Selective isolation of gold facilitated by second-sphere coordination with α-cyclodextrin Gold recovery using environmentally benign chemistry is imperative from an environmental perspective. Here we report the spontaneous assembly of a one-dimensional supramolecular complex with an extended {[K(OH 2 ) 6 ][AuBr 4 ] (α-cyclodextrin) 2 } n chain superstructure formed during the rapid co-precipitation of α-cyclodextrin and KAuBr 4 in water. This phase change is selective for this gold salt, even in the presence of other square-planar palladium and platinum complexes. From single-crystal X-ray analyses of six inclusion complexes between α-, β- and γ-cyclodextrins with KAuBr 4 and KAuCl 4 , we hypothesize that a perfect match in molecular recognition between α-cyclodextrin and [AuBr 4 ] − leads to a near-axial orientation of the ion with respect to the α-cyclodextrin channel, which facilitates a highly specific second-sphere coordination involving [AuBr 4 ] − and [K(OH 2 ) 6 ] + and drives the co-precipitation of the 1:2 adduct. This discovery heralds a green host–guest procedure for gold recovery from gold-bearing raw materials making use of α-cyclodextrin—an inexpensive and environmentally benign carbohydrate. The interaction of human beings with gold is an activity that has been ongoing since ancient times as a result of this precious metal’s unique physical and chemical properties. As the price of gold has skyrocketed during the past decade, a significant economic incentive exists for its recovery [1] , not only from ores, but also from the waste products of consumer electronics. In addition to this incentive, developing green methodologies for gold extraction and recovery is important from an environmental perspective. The most commonly used process for gold recovery involves the use of highly poisonous inorganic cyanides to convert gold(0) into a water-soluble Au(CN) 2 − coordination complex by a process known as leaching, followed by its isolation using cementation, absorption or solvent extraction as typical methods [2] . As application of cyanide leaching to gold recovery has often resulted [1] in contamination of the environment from accidental leakages and exposures, developing processes for gold recovery using environmentally benign chemistry is not only important from a green chemistry point of view, but it may also lead to procedures which will become more economically viable than the current ones. The use of host–guest chemistry [3] , which has the advantage of requiring only mild conditions in order to afford complexes with well-defined and specific non-covalent bonding interactions driving their recognition processes, has not been well investigated as an isolation procedure for gold. Some of the most common hosts are the cyclodextrins (CDs), which are cyclic oligosaccharides with hydrophobic cavities that can house nonpolar guests. They often lead to the formation of one-dimensional supramolecular inclusion polymers [4] , [5] , [6] , [7] , [8] , [9] , typically pseudopolyrotaxanes, with a wide variety of organic [10] , [11] , [12] , organometallic [13] , [14] , [15] , [16] , [17] , [18] , [19] and inorganic [20] , [21] , [22] , [23] guests. The structural compatibility between the CDs and the guests is the key preorganization parameter to consider when designing CD inclusion complexes, while hydrophobic interactions [24] , in addition to second-sphere coordination [25] , [26] , [27] , provide major contributions to the stabilities of these complexes. Although numerous single-crystal superstructures [4] , [5] , [6] , [7] , [20] of CD inclusion complexes exist in the literature, the formation of CD host–guest complexes with gold salts as guests has not been explored to our knowledge. Herein, we report the unprecedented and rapid formation of a well-defined one-dimensional single-crystalline material, which features a high-aspect-ratio and coaxial core-shell superstructure. It relies on the self-assembly of KAuBr 4 and α-CD in aqueous solution to form ( Fig. 1 ), as a co-precipitate, a 1:2 complex, KAuBr 4 ·(α-CD) 2 ( α·Br ), with an extended {[K(OH 2 ) 6 ][AuBr 4 ] (α-CD) 2 } n chain superstructure. The formation of this hybrid material is confirmed by scanning (SEM), transmission (TEM) electron and atomic force (AFM) microscopies, as well as by electron diffraction, while the superstructure has been characterized by single-crystal and powder X-ray diffraction (XRD). The rapid co-precipitation of the α·Br complex between KAuBr 4 and α-CD is highly specific: it does not materialize, for example, even if KAuCl 4 is employed as an alternative gold salt, or if β- or γ-CD is substituted for α-CD. We have also discovered that the co-precipitation of α·Br is selective for gold, even in the presence of other square-planar noble metal complexes, such as those involving palladium and platinum. A laboratory scale gold recovery process has also been developed, based on the selective co-precipitation of α·Br , by employing gold-bearing scraps as raw materials. From a detailed analysis of the single-crystal X-ray superstructures of an extensive range of inclusion complexes between α-, β- or γ-CDs with KAuX 4 (X=Cl, Br), we hypothesize that the perfect molecular recognition between the α-CD ring and the square-planar [AuBr 4 ] − anion, which leads to an axial orientation of the anion with respect to the channel of α-CD rings, facilitates a highly specific second-sphere coordination involving, not only the [AuBr 4 ] − anion, but also the [K(OH 2 ) 6 ] + cation, driving the formation and rapid selective co-precipitation of the α·Br complex. This bulk process, which is reminiscent [25] of the second-sphere coordination of transition-metal ammines with [18]crown-6, wherein [Cu(NH 3 ) 4 (H 2 O)][PF 6 ] 2 can be separated [28] as a crystalline co-precipitate from [Co(NH 3 ) 6 ][PF 6 ] 3 in aqueous solution, represents a promising strategy that relies on second-sphere coordination, providing a very attractive host–guest procedure for gold recovery in the form of KAuBr 4 , starting from gold-bearing raw materials and making use of α-CD, an inexpensive and environmentally benign carbohydrate, as the host. 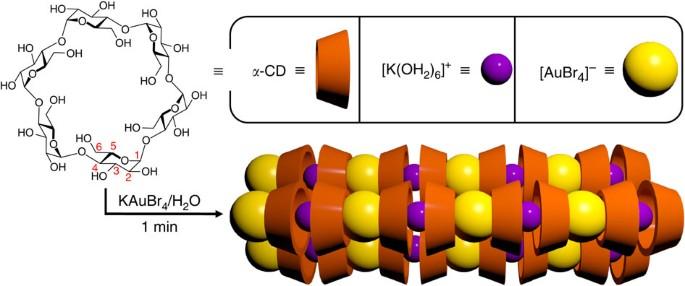Figure 1: Schematic representation of the spontaneous self-assembly of α·Br. Upon mixing KAuBr4and α-CD in water, a hydrogen-bonded linear superstructure forms spontaneously in <1 min. The cavities of the α-CDs oriented head-to-head, tail-to-tail form a continuous channel, which is filled by an alternating [K(OH2)6]+and [AuBr4]−polyionic chain to generate a cable-like superstructure that then tightly packs one with another (Supplementary Fig. S1) leading to crystals observable to the naked eye. Figure 1: Schematic representation of the spontaneous self-assembly of α·Br. Upon mixing KAuBr 4 and α-CD in water, a hydrogen-bonded linear superstructure forms spontaneously in <1 min. The cavities of the α-CDs oriented head-to-head, tail-to-tail form a continuous channel, which is filled by an alternating [K(OH 2 ) 6 ] + and [AuBr 4 ] − polyionic chain to generate a cable-like superstructure that then tightly packs one with another ( Supplementary Fig. S1 ) leading to crystals observable to the naked eye. Full size image Formation and characterization of α·Br Minimal variations in the building blocks employed in molecular self-assembly processes can lead to totally different superstructures and physical properties [29] , [30] , [31] , [32] , [33] , reflecting the subtle interplay between weak non-covalent bonding forces, particularly hydrogen bonding [34] , [35] , [36] , [37] in the case of CDs. Upon mixing any particular aqueous solution (20 mM, 1 ml) of KAuX 4 with any chosen aqueous solution (26.7 mM, 1.5 ml) of α-, β-, or γ-CDs at room temperature, a shiny pale brown suspension forms exclusively within a few minutes ( Fig. 2 and Supplementary Movie 1 ) when KAuBr 4 and α-CD form the 1:2 adduct, α·Br . Centrifugal filtration and drying under vacuum of the suspension permits the isolation of the α·Br complex in bulk as a pale brown powder. 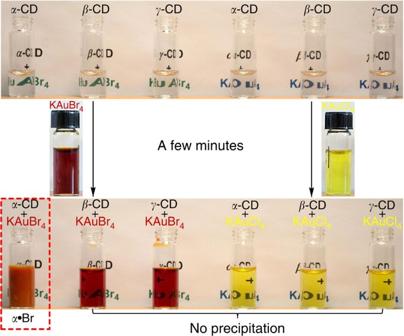Figure 2: Formation and co-precipitation of α·Br from KAuBr4and α-CD. When an aqueous solution (20 mM, 1 ml) of KAuX4(X=Cl or Br) is added to an aqueous solution (26.7 mM, 1.5 ml) of α-, β-, or γ-CD, a shiny pale brown suspension forms exclusively from the combination of KAuBr4and α-CD within 1–2 min (SeeSupplementary Movie 1). Figure 2: Formation and co-precipitation of α·Br from KAuBr 4 and α-CD. When an aqueous solution (20 mM, 1 ml) of KAuX 4 (X=Cl or Br) is added to an aqueous solution (26.7 mM, 1.5 ml) of α-, β-, or γ-CD, a shiny pale brown suspension forms exclusively from the combination of KAuBr 4 and α-CD within 1–2 min (See Supplementary Movie 1 ). Full size image SEM of an air-dried aqueous suspension of the α·Br complex reveals ( Fig. 3a ) the formation of long, needle-like crystals with extremely high aspect ratios. Examination of a suspension of these nanostructures by TEM reveals ( Fig. 3b ) that they have diameters of a few hundred nanometres and lengths on the order of micrometres. The nanostructures were stabilized under cryo-TEM conditions and then subjected to selected area electron diffraction (SAED). SAED patterns of the assembly of the α·Br complex show ( Fig. 3c ) clear and symmetrical diffraction spots, an observation which confirms the crystalline nature of the nanostructures. Although SEM and TEM can provide details of the morphology of α·Br , more detailed atomic-level structural information is required in order to understand the non-covalent bonding forces driving this highly selective molecular self-assembly process. 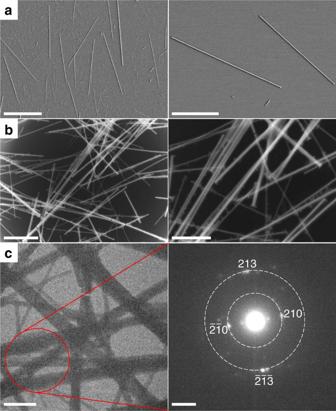Figure 3: Morphology of the nanostructures of α·Br. (a) SEM images of a crystalline sample prepared by spin-coating an aqueous suspension ofα·Bronto a silicon substrate, and then air-drying the suspension. (b) TEM images ofα·Brprepared by drop-casting an aqueous suspension ofα·Bronto a specimen grid covered with a thin carbon support film and air-dried. (c) Cryo-TEM image (left) and SAED pattern (right) of the nanostructures ofα·Br. As the selected area includes several crystals with different orientations and the crystals are so small that the diffraction intensities are relatively weak, we can assign the diffraction rings composed of diffraction dots but not the specific angles between different diffraction dots from the same crystal. The scale bars inaandbare 25 (left), 5 (right), 10 (left), 5 μm (right) and incare 1 μm (left) and 1 nm−1(right), respectively. Figure 3: Morphology of the nanostructures of α·Br. ( a ) SEM images of a crystalline sample prepared by spin-coating an aqueous suspension of α·Br onto a silicon substrate, and then air-drying the suspension. ( b ) TEM images of α·Br prepared by drop-casting an aqueous suspension of α·Br onto a specimen grid covered with a thin carbon support film and air-dried. ( c ) Cryo-TEM image (left) and SAED pattern (right) of the nanostructures of α·Br . As the selected area includes several crystals with different orientations and the crystals are so small that the diffraction intensities are relatively weak, we can assign the diffraction rings composed of diffraction dots but not the specific angles between different diffraction dots from the same crystal. The scale bars in a and b are 25 (left), 5 (right), 10 (left), 5 μm (right) and in c are 1 μm (left) and 1 nm −1 (right), respectively. Full size image Co-crystallisation by slow vapour diffusion of i PrOH into a dilute aqueous solution of KAuBr 4 and α-CD afforded single crystals of α·Br , which were suitable for X-ray crystallography. In the single-crystal superstructure ( Fig. 4a–c ) of α·Br , two α-CD tori are observed to be held together by means of intermolecular hydrogen bonding between the secondary (2°) hydroxyl faces of adjacent α-CD tori, which adopt a head-to-head packing arrangement, forming a supramolecular dimer. The dimer also serves the role of a second-sphere coordination cavitand occupied by the hexaaqua K + ion, ([K(OH 2 ) 6 ] + ) which adopts an equatorially distorted octahedral geometry with very short K–O distances [38] , [39] ranging from 2.37(1) to 2.44(1) Å (average 2.39 Å). We surmise that this superstructure forms in order for the [K(OH 2 ) 6 ] + ion to match the confines of the α-CD dimer cavity. It has been shown [8] , [14] , [16] , [17] , [18] , [38] , [39] previously that a few metal complexes, such as [12]crown-4·KCl (ref. 39 ) and metallocenium salts [16] , [17] , [18] , can form second-sphere coordination adducts [25] , [26] , [27] with CDs. Although, generally speaking, naked K + ions are incorporated interstitially between CD columns and are directly first-sphere coordinated with the hydroxyl groups of the CDs [9] , [40] , [41] , [42] , [43] , [44] , [45] , [46] , [47] , examples of hydrophilic fully hydrated K + ions encapsulated in the hydrophobic CD channels by means of second-sphere coordination are rare. The water molecules aligned along the c -axis direction of the octahedral [K(OH 2 ) 6 ] + ion are located statistically between the two symmetrical sites with 50:50 occupancies, which are related by an ~7° tilt about the c -axis. The square-planar [AuBr 4 ] − ions, centered between the primary (1°) hydroxyl faces of α-CD ( A ) and the adjacent α-CD ( B ), are disordered over two orientations with 50:50 occupancies and related by an ~9° rotation about the c -axis. Both α-CD tori A and B of the dimers in α·Br are distorted elliptically and elongated along the [AuBr 4 ] − planes with reference to the glycosidic ring O atoms. Although it was not possible to locate the H atoms associated with the H 2 O molecules on the [K(OH 2 ) 6 ] + ion, the distances between the c -axial Br and O atoms, which are 3.35(1) and 3.39(1) Å, are comparable with the mean value of 3.339(7) Å reported by Steiner [48] , an observation which suggests the presence of the significant c -axial [O−H···Br−Au] hydrogen bonding interactions ( Supplementary Table S4 ). All four Br atoms are close to twelve H5 and H6 atoms on the primary (1°) faces of the glucopyranosyl rings ( Fig. 1 ), with [C−H···Br−Au] contacts ( Supplementary Table S3 ) of 2.92−3.19 Å. The [C−H···Br−Au] hydrogen bonds [13] , [49] , [50] , [51] favour an equal distribution of orientations of the [AuBr 4 ] − anions around the c -axis. Accordingly, the dimers are stacked along the c -axis with [AuBr 4 ] − anions acting as linkers through multiple [C−H···Br−Au] hydrogen bonds with the α-CDs in the a − b plane and two [O−H···Br−Au] hydrogen bonds with the [K(OH 2 ) 6 ] + ions oriented in the c -axial direction. These α-CD dimers form parallel channels filled with [K(OH 2 ) 6 ] + cations and [AuBr 4 ] − anions, which line up in an alternating fashion to generate an infinite inorganic polyionic chain. This infinite cable-like supramolecular polymer can be dissected ( Fig. 4d ) structurally into head-to-head hydrogen-bonded α-CD dimers oriented tail-to-tail with respect to each other, forming an outer sheath-like organic nanotube with a coaxial, inorganic polyionic, inner chain, core. Bundles of these nanostructures are then tightly packed through hydrogen bonding between columns to form a well-ordered array that constitutes the single crystal. 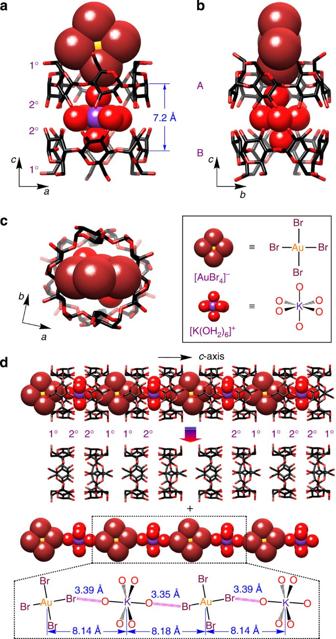Figure 4: Single-crystal X-ray structure of α·Br. The structure has the formula {[K(OH2)6][AuBr4](α-CD)2}n. (a) Side-on view showing the orientation of the primary and secondary faces of the α-CD rings in the extended structure. (b) Side-on view illustrating the second-sphere coordination of the [K(OH2)6]+ion with the [AuBr4]−ion. (c) Top view of the arrangement of the [AuBr4]−ion inside the cavity of α-CD. (d) Schematic illustration of the one-dimensional nanostructure extending along thec-axis in which the α-CD tori form a continuous channel occupied by alternating [K(OH2)6]+and [AuBr4]−ions. Hydrogen atoms areomitted for clarity. C, black; O, red; Br, brown; Au, yellow; K, purple. Hydrogen bonds are depicted as purple dash lines. Figure 4: Single-crystal X-ray structure of α·Br. The structure has the formula {[K(OH 2 ) 6 ][AuBr 4 ] (α-CD) 2 } n . ( a ) Side-on view showing the orientation of the primary and secondary faces of the α-CD rings in the extended structure. ( b ) Side-on view illustrating the second-sphere coordination of the [K(OH 2 ) 6 ] + ion with the [AuBr 4 ] − ion. ( c ) Top view of the arrangement of the [AuBr 4 ] − ion inside the cavity of α-CD. ( d ) Schematic illustration of the one-dimensional nanostructure extending along the c -axis in which the α-CD tori form a continuous channel occupied by alternating [K(OH 2 ) 6 ] + and [AuBr 4 ] − ions. Hydrogen atoms areomitted for clarity. C, black; O, red; Br, brown; Au, yellow; K, purple. Hydrogen bonds are depicted as purple dash lines. Full size image In order to confirm that the nanostructure of α·Br , obtained as a co-precipitate by solution-phase synthesis, is in agreement with the superstructure present in the single crystal of α·Br , a centrifugally filtrated sample of the as-synthesized suspension of the supramolecular complex was analysed ( Supplementary Fig. S9a ) by powder XRD (PXRD). The experimental PXRD pattern matches very well with the simulated pattern based on the single-crystal X-ray data, suggesting that the superstructures present in the single crystal of α·Br and the co-precipitated nanostructure are one and the same. In other words, the solution-phase synthesized one-dimensional nanostructures of α·Br are composed of single-crystalline bundles of one-dimensional molecular-level, cable-like, complexes ( Fig. 4d ) with high aspect ratios. As solution-phase synthesis affords much smaller crystals, single-molecule imaging studies using AFM can provide dimensional information of the sample, such as its height, with subnanometre precision. In order to investigate the physical dimensions of the self-assembled nanostructure formed between KAuBr 4 and α-CD on surfaces, a sample for AFM measurement was grown directly on the substrate. A droplet of a very dilute aqueous solution of KAuBr 4 (0.5 mM) and α-CD (1 mM) was spin-coated on freshly cleaved mica and dried under ambient conditions. The AFM image reveals ( Fig. 5a ) that the individual nanoassemblies have lengths on the order of several hundred nanometres and an average height ( Fig. 5b ) of 1.3±0.2 nm, which is consistent with the external diameter (~1.4 nm) of α-CD ( Fig. 5c ). These experiments provide insight into the mechanism of the molecular self-assembly process whereby these single-molecule-wide nanostructures are intermediates in the formation of the larger crystals observed by SEM and TEM. 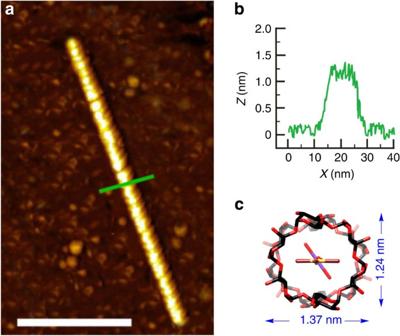Figure 5: AFM analysis of α·Br on a mica surface. (a) AFM image of a spin-coated sample ofα·Bron a freshly cleaved mica surface. (b) The cross-sectional analysis of (a). (c) Dimensions of the cross-section of the one-dimensional α-CD channel inα·Br. Scale bar, 100 nm. Figure 5: AFM analysis of α·Br on a mica surface. ( a ) AFM image of a spin-coated sample of α·Br on a freshly cleaved mica surface. ( b ) The cross-sectional analysis of ( a ). ( c ) Dimensions of the cross-section of the one-dimensional α-CD channel in α·Br . Scale bar, 100 nm. Full size image Insight into the spontaneous co-precipitation of α·Br It would appear that the spontaneous co-precipitation of the one-dimensional nanostructure of α·Br is highly selective as no similar phenomenon was observed from the other five combinations between KAuX 4 salts (X=Cl or Br) with α-, β- and γ-CDs. In order to gain insight into the mechanism behind the formation of the nanostructure of α·Br and the reason for its rapid co-precipitation, single crystals ( Supplementary Table S1 and Supplementary Figs S2−S7 ) of a series of inclusion complexes KAuCl 4 ·(α-CD) 2 ( α·Cl ), KAuBr 4 ·(β-CD) 2 ( β·Br ), KAuCl 4 ·(β-CD) 2 ( β·Cl ), KAuBr 4 ·(γ-CD) 3 ( γ·Br ), and KAuCl 4 ·(γ-CD) 3 ( γ·Cl ) were grown employing similar slow vapour diffusion methods and subjected to single-crystal XRD analysis. In contrast to α·Br , which adopts the orthorhombic space group P 2 1 2 1 2 ( Supplementary Fig. S1 ), the crystal structure ( Supplementary Fig. S2 ) of α·Cl is in the monoclinic ( β =90.041(4)°) space group P 2 1 . Both α-CD tori of the dimers in α·Br and α·Cl are elliptically distorted and elongated along the [AuX 4 ] − planes with respect to the glycosidic ring O atoms ( Supplementary Fig. S3 ). A significant difference in the role exhibited by the K + ion was observed between α·Br and α·Cl . In α·Cl , the K + ion is located outside the dimer cavity and enters into first-sphere coordination with seven primary hydroxyl groups belonging to two adjacent CD dimers. This observation suggests that the role of the K + ion is to act as a linker between adjacent CD dimers along the b -axis direction in α·Cl instead of acting as an isolated [K(OH 2 ) 6 ] + guest inside the CD dimer cavity in α·Br . The bridging of the K + ions in α·Cl along the b -axis results in the formation of one-dimensional coordination polymer chains composed of alternating α-CD dimers and K + ions, which then stack alternatively with [AuCl 4 ] − along the a -axis to constitute an extended two-dimensional superstructure ( Supplementary Fig. S8a ). In order to compare the orientation of the square-planar anions [AuBr 4 ] − and [AuCl 4 ] − in the CD channel, we define (i) the rotation angle of the [AuX 4 ] − anion viewed from the front ( Fig. 6 ) as φ , and (ii) the inclination angle of the [AuX 4 ] − anion viewed from the side with respect to the central axis of the CD tori ( Fig. 6 ) as θ . The [AuBr 4 ] − anion in α·Br has an orientation with φ =9.2° and θ =2.6°, whereas the [AuCl 4 ] − anion in α·Cl has a more tilted orientation with φ =17.1° and θ =2.6°. All the differences in superstructure between α·Br and α·Cl , as well as the unique spontaneous co-precipitation of α·Br , can be ascribed to the subtle size differences between the [AuBr 4 ] − and [AuCl 4 ] − anions. It is crucial to note that the average Au−Br bond length of 2.42 Å in α·Br is only 0.15 Å longer than the average Au−Cl bond length of 2.27 Å in α·Cl ( Supplementary Table S2 ). This observation highlights the fact that the longer bond length in [AuBr 4 ] − facilitates the second-sphere coordination of α-CD to [K(OH 2 ) 6 ] + and [AuBr 4 ] − , giving rise to the formation of α·Br and its unique superstructure. In addition, this second-sphere coordination results in the encapsulation of [K(OH 2 ) 6 ] + cations inside the cavities of the α-CD dimers, which we hypothesize restricts solvation of [K(OH 2 ) 6 ] + cations by water molecules from the bulk—the reason for the observed rapid co-precipitation. 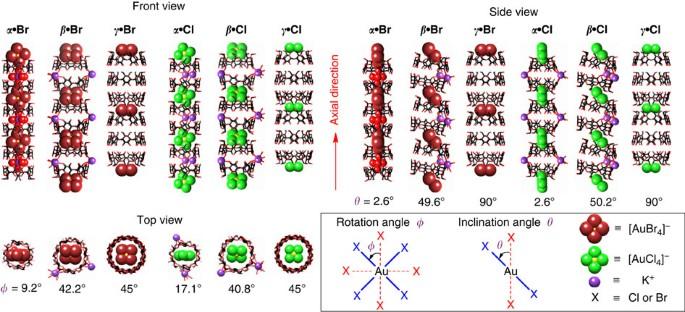Figure 6: Single-crystal superstructures of α·Br, α·Cl, β·Br, β·Cl, γ·Br and γ·Cl. The rotation angle of the [AuX4]−anion viewed from the front is defined asφ, and the inclination angle of the [AuX4]−anion viewed from the side with respect to the central axis of the CD tori is defined asθ. C, black; O, red; Br, brown; Cl, green; Au, yellow; K, purple. Figure 6: Single-crystal superstructures of α·Br, α·Cl, β·Br, β·Cl, γ·Br and γ·Cl. The rotation angle of the [AuX 4 ] − anion viewed from the front is defined as φ , and the inclination angle of the [AuX 4 ] − anion viewed from the side with respect to the central axis of the CD tori is defined as θ . C, black; O, red; Br, brown; Cl, green; Au, yellow; K, purple. Full size image The β-CD complexes β·Br and β·Cl , as well as the γ-CD complexes γ·Br and γ·Cl , are all isomorphous, an observation which indicates that the subtle differences between [AuBr 4 ] − and [AuCl 4 ] − no longer result in significant changes in superstructure. The K + ions in β·Br and β·Cl have similar bridging roles as they do in α·Cl , while the K + ions in γ·Br and γ·Cl reside outside the CD channel and are disordered. The β-CD tori in β·Br and β·Cl form head-to-head dimers similar to those in α·Cl , whereas the γ-CDs in γ·Br and γ·Cl form head-to-tail/head-to-head trimeric repeating units. Moreover, β-CD dimers in β·Br and β·Cl form zig-zag two-dimensional layered superstructures ( Supplementary Fig. S8b and c ). One common feature which describes all six complexes are that the CD rings stack along the longitudinal axes with [AuX 4 ] − anions acting as bridges, which are located inside the CD channels and are supported between the primary faces of the adjacent CD rings by [C−H···X−Au] hydrogen bonds, forming one-dimensional superstructures. With the expansion in size ongoing from α- to γ-CD tori, the angle φ increases from 9.2 to 45° for [AuBr 4 ] − and from 17.1 to 45° for [AuCl 4 ] − , while the angle θ increases from 2.6 to 90° for [AuBr 4 ] − and [AuCl 4 ] − ( Fig. 6 ), respectively. We hypothesize that this trend of [AuX 4 ] − to lie flatter is to shorten the length of the [C−H···X−Au] hydrogen bonds as much as possible and so facilitates the formation of the most stable host–guest superstructures. Except for α·Br in which the CD channels are filled up by [K(OH 2 ) 6 ] + and [AuBr 4 ] − , the other five complexes demonstrate ( Fig. 6 ) ‘bamboo’-like superstructures with isolated empty capsules formed by CD channels segmented by [AuX 4 ] − , and the K + cations are not encapsulated by the CD cavities. We suspect that the superstructures for these fives complexes result in the exposure of the K + cations to water molecules from the bulk, keeping these complexes solvated, and hence restricting precipitation. Stability and porosity of all complexes In order to assess the stability of all six complexes after activation using supercritical CO 2 (refs 52 , 53 ) (see Methods), we first of all examined their thermal stabilities using thermogravimetric analysis (TGA). TGA traces ( Supplementary Fig. S10 ) for all complexes start to show significant weight loss at 150 °C, suggesting that the samples are fully evacuated, while thermal decomposition occurs at temperatures over 150 °C. In order to examine sample structural stability upon activation, PXRD analyses ( Supplementary Fig. S9 ) were carried out on as-synthesized and activated samples. The well-matched PXRD patterns of as-synthesized and activated samples of α·Br confirm that its superstructure remains intact upon activation despite the lack of first-sphere coordination of K + ions between CD dimers. Comparison of the PXRD patterns of as-synthesized and activated samples of α·Cl , β·Br and β·Cl confirms the stability and crystallinity of their superstructures, which are formed by hydrogen bonding and K + ion coordination, upon activation. In contrast to these three samples, the activated samples of γ·Br and γ·Cl were found to be amorphous by PXRD, an observation which indicates that the fully hydrogen-bonded structures of γ·Br and γ·Cl are unstable and collapse after activation in the absence of K + ion coordination. The surface areas and porosities of all complexes were examined by CO 2 adsorption at 273 K ( Supplementary Figs S11 and S12 ). The isotherm of α·Br reveals a poor uptake and a capacity of only 3.5 cm 3 g −1 at 1 bar, corresponding to a Bruhauer-Emmett-Teller (BET) surface area of 35 m 2 g −1 . This observation stands in sharp contrast to α·Cl , which shows a modest uptake ability of 23 cm 3 g −1 at 1 bar with a BET surface area of 210 m 2 g −1 . This not insignificant difference can be attributed to their structural dissimilarities, in that the isolated capsules formed by segmentation of α-CD channels with [AuX 4 ] − are empty in α·Cl , whereas they are filled up by [K(OH 2 ) 6 ] + in α·Br ( Fig. 6 ). β·Br and β·Cl have empty capsules, similar to those in α·Cl , and so also show modest uptakes and comparable BET surface areas (224 m 2 g −1 for β·Br and 138 m 2 g −1 for β·Cl ). Both γ·Br and γ·Cl exhibit very low uptakes and BET surface areas, as the activation turned them into amorphous powders [54] , as indicated by PXRD ( Supplementary Fig. S9 ). These results are consistent with our hypothesis that co-precipitation of α·Br is a result of the α-CD dimer cavities being filled—that is, the [K(OH 2 ) 6 ] + cations are encapsulated and restricted from solvation. Selective isolation of gold from gold-bearing raw materials The selective co-precipitation of α·Br between α-CD and KAuBr 4 has prompted us to investigate if the high selectivity of α-CD rings towards trapping [AuBr 4 ] − anions is also effective in the presence of other square-planar noble metal complexes, for example, [PtX 4 ] 2− and [PdX 4 ] 2− (X=Cl, Br). In an attempt to obtain an estimate of the separation efficiency, α-CD (0.2 mmol × 2) was added separately to (i) a solution (3 ml) containing KAuBr 4 (33 mM), K 2 PtBr 4 (26 mM, saturated) and K 2 PdBr 4 (33 mM) ( Mixture 1 ), and also to (ii) another solution (3 ml) of KAuBr 4 (33 mM), K 2 PtCl 4 (24 mM, saturated) and K 2 PdCl 4 (33 mM) ( Mixture 2 ), respectively. Pale brown precipitates formed in both solutions immediately after the addition. Both precipitates were filtered, and the filtrates were diluted and subjected to inductively coupled plasma optical emission spectroscopy (ICP-OES) elemental analysis to determine the residual amounts of Au, Pt and Pd remaining in the mother liquor. The separation percentages for Au, Pt and Pd in both mixtures are defined by comparing contents of Au, Pt and Pd in the two mixtures before and after addition of α-CD. The ICP-OES analysis results show ( Fig. 7 ) that 78.3% of Au in Mixture 1 and 77.8% of Au in Mixture 2 were separated out of solution, whereas <3% of Pt and Pd was removed from both mixtures, values which are within the error limit of the experiment. These results reveal that the capture of [AuBr 4 ] − ions by α-CD to form α·Br in Mixture 1 and Mixture 2 is a highly selective process even in the presence of other noble metals and augurs well for developing a low cost and environmentally benign procedure for the separation of gold from complex mixtures of similar metal salts. 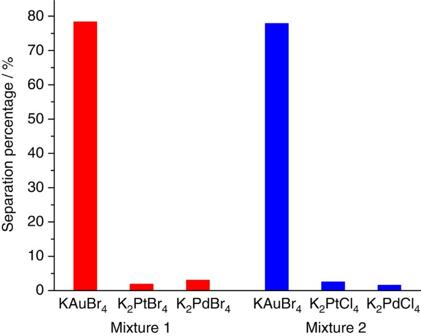Figure 7: Selective precipitation and separation of gold. The separation percentage, from mixtures 1 (red) and 2 (blue), is defined as (Cb−Ca)/Cb, whereCbandCaare the concentrations of each metal before and after addition of α-CD, respectively. Figure 7: Selective precipitation and separation of gold. The separation percentage, from mixtures 1 (red) and 2 (blue), is defined as ( C b − C a )/ C b , where C b and C a are the concentrations of each metal before and after addition of α-CD, respectively. Full size image In order to explore the practical potential of the selective co-precipitation of α·Br for gold recovery, we have employed gold-bearing scrap as the raw material to develop a laboratory scale gold recovery process. Taking into account that the pH of the [AuBr 4 ] − -bearing solution may vary in practice, we first of all studied the effect of pH on the co-precipitation of α-CD with [AuBr 4 ] − . Co-precipitation experiments conducted by adding α-CD into [AuBr 4 ] − solutions (50 mM) of various pH (1.4−5.9) indicate (see Methods and Supplementary Fig. S13 ) a trend in the residual concentration of [AuBr 4 ] − in the filtrate after filtration to remove the co-precipitates. When the pH is increased from 1.4 to 2.5, the residual concentration of [AuBr 4 ] − decreases to ~6.8 mM—which is consistent with the bulk solubility of α·Br in water—and remains constant at this value until pH 5.9 is attained. This result reveals that the co-precipitation of α-CD with [AuBr 4 ] − is dependent on pH, and that the pH range 2.5–5.9 is the suitable one to initiate this co-precipitation process. We have managed (see Fig. 8 and Methods) to convert two scrap gold-bearing alloys containing 58% wt of Au and 42% wt of other metals (Zn, Cu and Ag) into HAuBr 4 by dissolving them with a mixture of concentrated HBr and HNO 3 as the etchant solution. On the basis of this pH experiment, KOH was used to neutralize both dissolved gold solutions to pH 4–6, and consequently convert HAuBr 4 to KAuBr 4 . When α-CD was added to both solutions, the co-precipitation of α·Br occurred immediately, even in the presence of the significant amounts of Zn and Cu salts. The co-precipitated α·Br complex—namely, recovered gold—was separated from impurities by filtration and then reduced with a reductant, such as Na 2 S 2 O 5 , to afford the recovered gold metal. The residual gold in the filtrate can be recycled while α-CD can be reused by recrystallisation from the filtrate. This laboratory scale process is highly selective for gold, as well as being economic, fast and feasible. As it doesn’t involve the use of toxic inorganic cyanides, this process is much more environmentally benign in comparison with the universally accepted cyanidation process [2] . Further optimization of process conditions and parameters is ongoing in our laboratories. 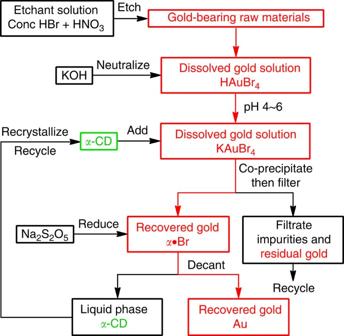Figure 8: Gold recovery process flow diagram. Red arrows indicate the flow direction of the gold recovery. Na2S2O5: Sodium metabisulfite. Figure 8: Gold recovery process flow diagram. Red arrows indicate the flow direction of the gold recovery. Na 2 S 2 O 5 : Sodium metabisulfite. Full size image The rapid solution-phase self-assembly of KAuBr 4 and α-CD leads to the formation of a host–guest complex ( α·Br ), which co-precipitates as needle-like crystals with a superstructure wherein α-CD nanochannels are filled up by [K(OH 2 ) 6 ] + and [AuBr 4 ] − ion pairs in an alternating fashion through multiple preorganized, hydrogen bonding interactions. The unique formation and co-precipitation of α·Br suggest that this self-assembly process arises as a consequence of the perfect structural correspondence between the stereoelectronics associated with [K(OH 2 ) 6 ] + , [AuBr 4 ] − and α-CD. The axial [O−H···Br−Au] and the equatorial [C−H···Br−Au] hydrogen bonding-triggered second-sphere coordination has an indispensible role in governing the formation of α·Br and its rapid co-precipitation. A fundamental understanding of these multiple non-covalent bonding phenomena provides insight into the nature of the molecular self-assembly processes, wherein extremely subtle changes in substrates lead to different superstructures and properties. This specific co-precipitation procedure establishes a motif for the selective capture of gold in the form of KAuBr 4 , starting from gold-bearing raw materials and mixtures of six square-planar anions ([AuX 4 ] − , [PtX 4 ] 2− and [PdX 4 ] 2− , X=Cl, Br). The research highlights the potential application of a green technology for an economic recovery process of gold by using the inexpensive and environmentally benign α-CD. Materials Chemicals were purchased as reagent grade from Aldrich and used without further purification. High purity water was generated by a Milli-Q apparatus (Millipore). Formation and characterization of α·Br An aqueous solution of KAuBr 4 (25 mM, 1 ml) was added to an aqueous solution of α-CD (50 mM, 1 ml) at room temperature. A glossy pale brown suspension formed within a few minutes of shaking. Centrifugal filtration and drying under vacuum of the suspension allows isolation of the α·Br complex as a pale brown powder in ~70% yield. The phase purity of this complex was confirmed ( Supplementary Fig. S9a ) by PXRD. The as-synthesized suspension was spin-coated on a silicon wafer and dried under air. SEM images were obtained using a Hitachi S-4800 FS-SEM. TEM images were obtained on a Hitachi H-2300 TEM operating at 80 kV. SAED patterns were taken with a Hitachi H-8100 instrument at a temperature of 113 K. Powder XRD data were collected on a Rigaku ATXG X-ray diffractometer using Cu-K α radiation ( λ =1.54178 Å, 50 kV, 240 mA) at room temperature. The observed intensities are in very good agreement with the calculated diffraction pattern based on the single-crystal data ( Supplementary Fig. S9a ). Crystallisations and X-ray analyses for all complexes For α·Br : Aqueous solutions of KAuBr 4 (3.33 mM, 1 ml) and α-CD (6.67 mM, 1 ml) were mixed together. For α·Cl , β·Br , β·Cl , γ·Br , and γ·Cl : Aqueous solutions of KAuX 4 (20 mM, 1 ml) and CDs (26.7 mM, 1.5 ml) were mixed together and passed through a Pall syringe filter (pore size 0.45 μm) into culture tubes (6 × 50 mm). The tubes were allowed to stand at room temperature in a closed 20 ml scintillation vial containing EtOH or MeOH (5 ml). After about 1 week, the crystals, which appeared in the tubes, were selected and mounted using oil (Infineum V8512) on a glass fibre and transferred to the cold gas stream cooled by liquid N 2 on Bruker APEX-II CCDs (charge-coupled devices) with graphite monochromated Mo-K α or Cu-K α radiation. The structures were solved by direct methods and refined subsequently using OLEX2 software. CCDC 918412−918417 contain the supplementary crystallographic data for this article. These data can be obtained free of charge from the Cambridge Crystallographic Data Centre via www.ccdc.cam.ac.uk/data_request/cif . AFM Measurements Tapping mode AFM measurements were performed using a multimode scanning probe microscope with a Nanoscope 3A controller (Digital Instruments, Veeco Probes), operating at room temperature in air. AFM images were recorded on freshly cleaved mica surfaces (Ruby Muscovite mica, SJ Mica & Trading), prepared by spin-coating a droplet of a very dilute aqueous solution of KAuBr 4 (0.5 mM) and α-CD (1 mM) and dried in a chemical hood at room temperature. AFM studies were executed with a microfabricated ultrasharp silicon cantilever (model NSG-01, NT-MDT Co.) using the tapping mode at their resonant frequency (149 kHz), having a spring constant of 5 N m −1 and a normal tip radius of ~10 nm. AFM images were recorded at scan frequencies of 1−2 Hz with minimal loading forces applied and optimized feedback parameters. Several images were obtained at separate locations across the mica surfaces to ensure a high degree of reproducibility of the recorded molecular nanostructures. All the images consist of 512 × 512 pixels and were analysed by means of Nanoscope 5.12r5 software. The width of the nanostructure of α·Br was corrected owing to the tip convolution by taking into account a tip radius of 10 nm and the height of the nanostructure of 1.3±0.2 nm, determined from the topographical profile, we estimate a corrected width of ~1.4 nm. TGA Measurements TGA experiments were performed on a Mettler Toledo TGA/DSC 1 Star e System (Schwerzenbach, Switzerland) interfaced with a PC using Star e software (version 9.10). Samples were placed in alumina pans and heated at a rate of 10 °C min −1 from 25 to 800 °C under a nitrogen atmosphere. Gas adsorption experiments Supercritical CO 2 drying was performed using a Tousimis Samdri PVT-30 critical point dryer (Tousimis, Rockville, MD, USA). CO 2 isotherm measurements were carried out on an Autosorb-1MP instrument (Quantachrome Instruments, Boynton Beach, FL). Measurements were performed at 273 K and were held constant using a Polyscience recirculating chiller (PolyScience, Niles, IL). After filtering the sample, it was transferred into a Tousimis Samdri-PVT-three-dimensional super-critical CO 2 dryer. The temperature was lowered to 0 °C, and the chamber was filled with liquid CO 2 (ultrahigh grade CO 2 with a siphon from Air-Gas Inc., was used). The sample was soaked for 8 h in total, venting for 5 min every 2 h. The chamber was then heated to 40 °C, and the supercritical CO 2 was bled off at a rate of 1 ml min −1 until the chamber reached ambient pressure (~12 h). The chamber was opened and the sample was quickly sealed and taken into an argon atmosphere glove box for further manipulations. The dried sample was transferred into a preweighed glass sample tube which was sealed and quickly transferred to a system providing 10 −4 torr dynamic vacuum. The sample was kept under vacuum at room temperature for 18 h and was then used for CO 2 adsorption measurements. After measurement, the sample was returned to the argon atmosphere glove box and a final mass was calculated. ICP-OES analyses ICP-OES was carried out on a Varian ICP-OES spectrometer (Varian, Walnut Creek, CA) equipped with a CCD detector and argon plasma that cover the spectral range from 175 to 785 nm. The samples, filtered through a 0.45-μm Acrodisc, were diluted with ultrapure H 2 O and analysed for contents of Au, Pt and Pd as compared with standard solutions. pH experiments Seven [AuBr 4 ] − solutions (50 mM, 2 ml) with pH values of 1.4, 1.7, 1.8, 1.9, 2.5, 4.8 and 5.9 were prepared by neutralizing identical amounts of HAuBr 4 with different amounts of KOH in water. The pHs of these solutions were measured with a Hanna Checker pH metre. When α-CD (0.2 mmol × 7) was added to the above seven solutions, the co-precipitation occurred immediately. The co-precipitates were removed by filtration, and the filtrates were then diluted and analysed for their residual concentrations of [AuBr 4 ] − by ICP-OES. Process for gold recovery from gold-bearing materials A red gold alloy scrap (58% wt Au and 42% wt Cu and Ag, % wt Cu>Ag) and a yellow gold alloy scrap (58% wt Au and 42% wt Cu, Zn and Ag, % wt Ag>Cu>Zn) were employed as gold-bearing raw materials to explore a laboratory scale gold recovery process. General procedure ( Fig. 8 ): the gold-bearing raw material (250 mg) was dissolved in a mixture (4 ml) of concentrated HBr and HNO 3 (3/1, V/V). Then, the dissolved gold solution was neutralized to pH 4–6 with KOH and filtered to remove insoluble silver bromide. When α-CD (1.48 mmol, 1.44 g) was added to the solution, the co-precipitation of α·Br occurred immediately. Co-precipitated α·Br —namely, recovered gold—was separated by filtration. The residual gold in the filtrate can be recycled with the next process. The solid-state α·Br was dispersed into water, and then reduced with Na 2 S 2 O 5 (300 mg) to give the recovered gold metal as a precipitate. The recovered gold metal was collected by decanting off the aqueous, and the remaining α-CD in the liquid phase recycled by recrystallisation. For the red gold alloy scrap sample, the recovered gold was obtained in 89% yield and 97% purity (ICP-OES). For the yellow gold alloy scrap sample, the recovered gold was obtained in 92% yield and 95% purity (ICP-OES). Accession codes: The single-crystal diffraction data for all six complexes were deposited in the Cambridge Crystallographic Data Centre (CCDC) and the deposition numbers are CCDC 918412−918417. How to cite this article: Liu, Z. et al . Selective isolation of gold facilitated by second-sphere coordination with α-cyclodextrin. Nat. Commun. 4:1855 doi: 10.1038/ncomms2891 (2013).